High-efficiency direct methane conversion to oxygenates on a cerium dioxide nanowires supported rhodium single-atom catalyst Direct methane conversion (DMC) to high value-added products is of significant importance for the effective utilization of CH 4 to combat the energy crisis. However, there are ongoing challenges in DMC associated with the selective C−H activation of CH 4 . The quest for high-efficiency catalysts for this process is limited by the current drawbacks including poor activity and low selectivity. Here we show a cerium dioxide (CeO 2 ) nanowires supported rhodium (Rh) single-atom (SAs Rh-CeO 2 NWs) that can serve as a high-efficiency catalyst for DMC to oxygenates (i.e., CH 3 OH and CH 3 OOH) under mild conditions. Compared to Rh/CeO 2 nanowires (Rh clusters) prepared by a conventional wet-impregnation method, CeO 2 nanowires supported Rh single-atom exhibits 6.5 times higher of the oxygenates yield (1231.7 vs. 189.4 mmol g Rh −1 h −1 ), which largely outperforms that of the reported catalysts in the same class. This work demonstrates a highly efficient DMC process and promotes the research on Rh single-atom catalysts in heterogeneous catalysis. Methane (CH 4 ) is in fact among the most important and attractive feedstocks for producing methanol (CH 3 OH) and other high value-added products in the chemical industry [1] , [2] . In the traditional processes, CH 4 is converted into CH 3 OH indirectly via the formation of syngas (H 2 and CO), which is an energy-hungry process that needs to be performed under high temperature [3] , [4] . Therefore, the direct CH 4 conversion (DMC) to CH 3 OH, which is regarded as a “dream reaction” in chemical industry, has been the subject of intensive study for decades [5] , [6] , [7] . For instance, Periana et al. reported that CH 4 can be converted to CH 3 OH by mercuric ions in the presence of concentrated sulfuric acid [8] . Sushkevich et al. [9] synthesized a copper-containing zeolite catalyst and used it for the conversion of CH 4 to CH 3 OH with high selectivity (~ 97%) at 200 °C. More recently, Agarwal et al. used colloidal gold–palladium nanoparticles (Au–Pd NPs) to catalyze the DMC to CH 3 OH, methylhydroperoxide (CH 3 OOH), and formic acid (HCOOH) in the presence of hydrogen peroxide (H 2 O 2 ) and oxygen (O 2 ) [10] . The yield of these primary oxygenates product reaches ~53.6 mol kg cat −1 h −1 at a selectivity of 88.0% at 50 °C [10] . Shan et al. [2] reported that mononuclear rhodium species on ZSM-5 can catalyze DMC to CH 3 OH and acetic acid (CH 3 COOH) using O 2 and carbon monoxide (CO) with the total yield of oxygenates ~10 mmol g cat. −1 h −1 and the selectivity of CO 2 ~ 15% [2] . Despite the tremendous progress on the development of catalysts and technologies, DMC to oxygenates is extremely challenging because the selective activation of C−H bonds in CH 4 under mild conditions is a tough issue. It is thus highly desired to develop active and selective catalysts for the DMC to oxygenates. Noble metals-based single-atom catalysts (SACs) have emerged as a new frontier in heterogenous catalysis because of large ratio of surface atoms, low-coordination environment of metal centers, and strong metal–support interactions [11] , [12] , [13] . They have been widely studied in diverse processes with superior catalytic performance, including CO oxidation, CH 4 conversion, oxygen reduction, water gas shift reaction, and so on [14] , [15] , [16] . Recent investigations show that SACs can be used as highly active and selective catalysts for alkynes hydrogenation, in which the isolated active sites are geometrically in favor of the selective hydrogenation of alkynes [17] , [18] , [19] , [20] . For instance, Kyriakou et al. [17] demonstrated that the isolated Pd atoms in a Cu surface can be used as a highly selective catalyst for the hydrogenation of styrene and acetylene as compared with pure Cu or Pd metal. Yan et al. [18] claimed that Pd SAs can selectively catalyze butadiene to butene because of the mono-π-adsorption mode and the steric effect induced by butadiene adsorption on the isolated Pd atoms. Typical for CH 4 conversion, Tang et al. [15] reported that the single-site Rh 1 O 5 anchored in microporous aluminosilicates (ZSM-5) can catalyze the DMC to CH 3 COOH and CH 3 OH in the presence of CH 4 , CO, and O 2 at ≤ 150 °C. It is found that the single-site Rh 1 O 5 plays the role of the active site for DMC, while the rhodium oxide NPs on ZSM-5 are even not active for this transformation [15] . Kwon et al. [16] demonstrated that Rh SA on ZrO 2 can be used for the DMC to CH 3 OOH and CH 3 OH in H 2 O 2 solution at 70 °C. However, the selectivity of oxygenates from Rh SA on ZrO 2 is ~ 70% due to the different decomposition rate of H 2 O 2 and CH 3 OOH on ZrO 2 [16] . Inspired by these reports, we believe that the Rh SACs can be used as promising catalysts for DMC, and the selectivity of oxygenates may be strongly related to the support for anchoring Rh SA. Herein, we synthesized Rh-based SACs on CeO 2 nanowires (SAs Rh-CeO 2 NWs) via a simple hydrothermal process. The results show that SAs Rh-CeO 2 NWs can be used as a highly efficient catalyst for DMC to oxygenates in the presence of H 2 O 2 at 50 °C. Different from the previous work, our work reveals that the support for anchoring Rh SAs (i.e., CeO 2 NWs) is involved in the formation of radicals, which can further enhance the activity of DMC. The total yield and selectivity of oxygenates reach ~1231.7 mmol g Rh −1 h −1 and 93.9%, respectively. To the best of our knowledge, the current DMC performance outperforms the reported catalysts in literatures. In situ characterizations and theoretical calculations show that CeO 2 NWs play a vital role in the formation of ∙OOH and ∙OH radicals. SAs Rh-CeO 2 NWs can selectively activate CH 4 to ∙CH 3 , which further combines with ∙OOH and ∙OH radicals to form CH 3 OH and CH 3 OOH, respectively. By contrast, the Rh/CeO 2 NWs tend to overoxidize CH 4 to CO x species with the assistance of ∙OH, leading to a low oxygenates’ yield and selectivity (189.4 mmol g Rh −1 h −1 and 56.4%). Preparation and morphology characterization CeO 2 NWs were prepared via a simple hydrothermal process by adding cerium chloride (CeCl 3 ), sodium oleate, deionized water (H 2 O), and n -butylamine into a stainless reactor. The synthetic method of SAs Rh-CeO 2 NWs was the same as that of CeO 2 NWs, except for adding additional sodium hexachlororhodate (Na 3 RhCl 6 ). Rh/CeO 2 NWs and Rh/CeO 2 -com were prepared by impregnating Na 3 RhCl 6 on the as-prepared CeO 2 NWs and commercial CeO 2 via a conventional wet-impregnation method. 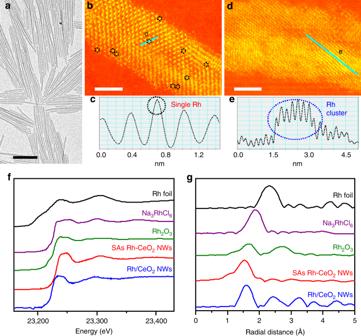Fig. 1: Structural analyses of SAs Rh-CeO2NWs and Rh/CeO2NWs. aTEM image of the SAs Rh-CeO2NWs.bAC-HAADF/STEM image in temperature color of the SAs Rh-CeO2NWs. The isolated Rh atoms are marked with black circles.cThe intensity profile recorded from the line in panel (b).dAC-HAADF/STEM image in temperature color of the Rh/CeO2NWs. The Rh cluster is marked with blue line.eThe intensity profile recorded from the line in panel (d).f,gRh K-edge XANES spectra (f) and Rh K-edge EXAFS spectra inRspace (g) of the Rh foil, Na3RhCl6, Rh2O3, SAs Rh-CeO2NWs, and Rh/CeO2NWs. The scale bars in (a), (b), and (d) are 100, 2, and 2 nm, respectively. The physicochemical properties are listed in Supplementary Table 1 . Transmission electron microscopy (TEM) image shows that uniform CeO 2 NWs with a diameter and length of ~ 6.2 nm and ~ 260 nm are obtained (Supplementary Fig. 1 ). No Rh nanoparticles are observed in TEM image, indicating that Rh atoms are well dispersed in SAs Rh-CeO 2 NWs (Fig. 1a ). The aberration-corrected high-angle annular dark-field scanning transmission electron microscopy (AC-HAADF/STEM) image in temperature color of SAs Rh-CeO 2 NWs indicates Rh atoms are presented as SA state (Fig. 1b, c ; Supplementary Fig. 2 ). By contrast, Rh clusters with the size of ~1.5 nm appear in the AC-HAADF/STEM image in temperature color of Rh/CeO 2 NWs (Fig. 1d, e ; Supplementary Fig. 3 ). In X-ray diffraction (XRD) pattern of SAs Rh-CeO 2 NWs, only the characteristic peaks of CeO 2 at 2 θ = 28.5, 33.1, 47.5, 56.3, 69.4, 76.7, 79.1, and 88.4° (PDF No. 43-1002) are observed (Supplementary Fig. 4 ), indicating that Rh atoms are highly dispersed on CeO 2 NWs and commercial CeO 2 , despite the full wavelength at half maximum (FWHM) of the characteristic peaks corresponding to CeO 2 NWs is much broader than that of commercial CeO 2 due to its small diameter of ~6.2 nm [21] . It should be noted that the absence of peaks corresponding to Rh clusters in the XRD pattern of Rh/CeO 2 NWs might be attributed to the very small-sized Rh clusters and low content of Rh in the catalyst. X-ray photoelectron spectroscopy measurements were performed to characterize the chemical states of elements on the surface of CeO 2 NWs, SAs Rh-CeO 2 NWs, Rh/CeO 2 NWs, and Rh/CeO 2 -com. As shown in Supplementary Fig. 5 , it is found that Rh are in their oxidation state (Rh 3+ ), while Ce consist of Ce 4+ (881.8, 888.3, 897.6, 900.3, 907.2, and 916.0 eV) and Ce 3+ (884.6 and 903.1 eV) [22] . The binding energy shifts of Rh in XPS spectra indicate that the different synergies among those catalysts. Compared with the Rh/CeO 2 -com (308.9 eV) and Rh/CeO 2 NWs (309.1 eV), Rh 3d5/2 peak obviously shifts to 309.4 eV in SAs Rh-CeO 2 NWs, suggesting the existence of electron transfer from Rh to CeO 2 in SAs Rh-CeO 2 NWs (Supplementary Fig. 5a ). On the other hand, detailed peak fittings demonstrate that the proportions of Ce 3+ are different among these samples (Supplementary Fig. 5b ). In particular, the proportion of Ce 3+ in Rh/CeO 2 -com is 12.4%, which is much lower than that in CeO 2 NWs (16.0%), Rh/CeO 2 NWs (16.5%), and SAs Rh-CeO 2 NWs (16.7%). XPS results imply a much stronger synergy exists in SAs Rh-CeO 2 NWs in comparison with Rh/CeO 2 NWs and Rh/CeO 2 -com. No obvious peaks in Na 1 s and Cl 2p XPS spectra suggest that neglect amount of Na and Cl remain on catalysts (Supplementary Fig. 5c, d ). Fig. 1: Structural analyses of SAs Rh-CeO 2 NWs and Rh/CeO 2 NWs. a TEM image of the SAs Rh-CeO 2 NWs. b AC-HAADF/STEM image in temperature color of the SAs Rh-CeO 2 NWs. The isolated Rh atoms are marked with black circles. c The intensity profile recorded from the line in panel ( b ). d AC-HAADF/STEM image in temperature color of the Rh/CeO 2 NWs. The Rh cluster is marked with blue line. e The intensity profile recorded from the line in panel ( d ). f , g Rh K-edge XANES spectra ( f ) and Rh K-edge EXAFS spectra in R space ( g ) of the Rh foil, Na 3 RhCl 6 , Rh 2 O 3 , SAs Rh-CeO 2 NWs, and Rh/CeO 2 NWs. The scale bars in ( a ), ( b ), and ( d ) are 100, 2, and 2 nm, respectively. Full size image To study the electronic structures and coordination states of Rh in the SAs Rh-CeO 2 NWs and the Rh/CeO 2 NWs, X-ray absorption near-edge spectroscopy (XANES) and extended X-ray fine structure (EXAFS) were measured at Rh K-edge. Rh foil, Rh 2 O 3 , and Na 3 RhCl 6 were used as references. Comparing with the edge position in the XANES spectra of references, Rh in SAs Rh-CeO 2 NWs and Rh/CeO 2 NWs are presented as their oxidation states (Fig. 1f ). As shown in Fig. 1g , the Rh−Rh coordination, Rh−Cl coordination, Rh−O, and the second shell of Rh−O coordination are observed at ~2.3 Å, ~1.9 Å, ~1.7 Å, and ~2.7 Å, respectively [15] . For Rh/CeO 2 NWs, Rh−O, and Rh−Rh coordination appear at ~1.6 Å and ~2.4 Å in the R -space EXAFS spectrum, indicating the presence of Rh clusters in Rh/CeO 2 NWs. By contrast, only the feature of Rh−O coordination at ~1.6 Å is observed in the R -space spectrum of SAs Rh-CeO 2 NWs (Fig. 1g ). The disappearance of Rh−Rh coordination implies that Rh atoms in SAs Rh-CeO 2 NWs are presented as isolated atoms, which is in good agreement with the observations in AC-HAADF/STEM image [16] , [23] . It is noted that no obvious Rh−Cl coordination is observed in the EXAFS spectrum of SAs Rh-CeO 2 NWs, indicating that the Rh atoms are anchored by O atoms in CeO 2 NWs via Rh−O coordination. In addition, the structures of SAs Rh-CeO 2 NWs and Rh/CeO 2 NWs were verified by the diffuse reflectance-infrared Fourier transform spectroscopy (DRIFTS) measurement using CO as a probe. As shown in Supplementary Fig. 6a , different from the previous reports that Rh SA gives geminal peaks in 2000−2100 cm −1 , only one broad and weak peak is observed at 2000−2150 cm −1 in the CO-DRIFTS spectrum of SAs Rh-CeO 2 NWs, which may be attributed to the low CO coverage on SAs Rh-CeO 2 NWs [24] . The presence of oxidation species at 1250−1700 cm −1 indicates that the adsorbed CO molecules are oxidized, further confirming the low CO coverage on the surface of SAs Rh-CeO 2 NWs. When SAs Rh-CeO 2 NWs was pretreated in CO at 50 °C for 0.5 h, the intensity of peak at 2000−2150 cm −1 obviously increases, despite the appearance of oxidation species. Further increasing the pre-treatment temperature to 150 °C, two intense peaks appear at 2101 and 2030 cm −1 in CO-DRIFTS spectrum of SAs Rh-CeO 2 NWs, which correspond to the symmetric and asymmetric vibration of gem-dicarbonyl doublet CO (i.e., Rh(CO) 2 ) (Supplementary Fig. 6a , red curve) [25] . For Rh/CeO 2 NWs, in addition to the peaks of oxidation species, multiple peaks corresponding to the symmetric (2101 cm −1 ) and asymmetric vibration (2030 cm −1 ) of Rh(CO) 2 and CO linear adsorption on Rh δ+ (2133 cm −1 ) are observed in CO-DRIFTS spectrum (Supplementary Fig. 6b ). When Rh/CeO 2 NWs was pretreated at 50 °C and then 150 °C for 0.5 h, two peaks appear at 1860 and 2060 cm −1 in CO-DRIFTS spectrum, which correspond to the CO bridge adsorption and linear adsorption on Rh, respectively (Supplementary Fig. 6b , red curve) [24] , [25] . The absence of CO bridge adsorption in the CO-DRIFTS spectrum further confirms the structures of Rh SA in SAs Rh-CeO 2 NWs, which is in good agreement with the result of AC-HAADF/STEM and X-ray absorption spectroscopy [25] . DMC performance of SAs Rh-CeO 2 NWs and Rh/CeO 2 NWs All the catalysts of Rh/CeO 2 -com, Rh/CeO 2 NWs, and SAs Rh-CeO 2 NWs were used for DMC in a pressurized reactor. Products were analyzed by gas chromatography and 1 H nuclear magnetic resonance spectroscopy ( 1 H-NMR). As shown in Fig. 2a , Rh/CeO 2 -com gives the CH 3 OH, CH 3 OOH, and CO x yield of 17.6, 15.6, and 137.4 mmol g Rh −1 h −1 , respectively. When Rh/CeO 2 NWs are used as a catalyst, the yield of CH 3 OH and CH 3 OOH increase to 170.4 mmol g Rh −1 h −1 and 19.0 mmol g Rh −1 h −1 , respectively, while the total yield of CO x is 146.3 mmol g Rh −1 h −1 . The low selectivities of oxygenate on Rh/CeO 2 -com (19.5%) and Rh/CeO 2 NWs (56.4%) indicate that CH 4 tends to be overoxidized into CO x on Rh/CeO 2 -com and Rh/CeO 2 NWs. By contrast, when SAs Rh-CeO 2 NWs are used as a catalyst, the selectivity of CO x significantly decreases to 6.1%, indicating that the overoxidation of CH 4 is strongly suppressed on SAs Rh-CeO 2 NWs. Correspondingly, the yield of CH 3 OH and CH 3 OOH significantly increase to 940.3 and 291.4 mmol g Rh −1 h −1 , respectively. Moreover, SAs Rh-CeO 2 NWs were tested for DMC under different conditions (i.e., temperature, H 2 O 2 concentration, CH 4 pressure, and catalysts amount). As depicted in Fig. 2b , it is found that the increase of temperature leads to a volcano-shape selectivity and yield of oxygenates. Typically, the selectivity and yield of oxygenates are 91.4% and 786.3 mmol g Rh −1 h −1 at 30 °C, which further increases to 93.9% and 1231.7 mmol g Rh −1 h −1 at 50 °C. Further increase in temperature will lead to a decrease in both the selectivity and yield of oxygenates. A similar tendency is observed when the concentration of H 2 O 2 is increased from 0.1 to 1.5 M (Fig. 2c ). For instance, the selectivity and yield of oxygenates are 67.1% and 145.0 mmol g Rh −1 h −1 at the H 2 O 2 concentration of 0.1 M, which significantly increase to 93.9% and 1231.7 mmol g Rh −1 h −1 at the H 2 O 2 concentration of 1.0 M, indicating H 2 O 2 can significantly promote the DMC activity. It is noted that a further increase of H 2 O 2 concentration to 1.5 M will result in a slight decay in oxygenates selectivity and yield. Furthermore, the effects of CH 4 partial pressure on DMC performance were studied. As shown in Fig. 2d , the selectivity of CO x strongly increases from 6.1% to 21.1% when the CH 4 partial pressure is increased from 0.5 MPa to 3 MPa, despite the similar yield of oxygenates. We thus further tested the DMC performance by altering the weight of the catalyst, as shown in Supplementary Fig. 7 . It is found that the yield of CH 3 OH and CH 3 OOH steadily increase as the increasing weight of catalyst, while the selectivity of CH 3 OH and CH 3 OOH are kept at ~94%. The positive effects of H 2 O 2 concentration and catalyst weight but negligible effects of CH 4 partial pressure on the oxygenates selectivity imply that Rh SA can efficiently activate C−H bonds in CH 4 under the optimized conditions, and the rate-determining steps solely involve the reaction of CH 4 activation intermediates with H 2 O 2 (Fig. 2; Supplementary Fig. 7 ) [10] . In addition, SAs Rh-CeO 2 NWs were used in ten consecutive DMC cycles to test the stability. As shown in Supplementary Fig. 8 , no obvious decays in oxygenates selectivity and yield are observed after ten consecutive DMC cycles. The structures of Rh SA are reserved in the spent SAs Rh-CeO 2 NWs, indicating that SAs Rh-CeO 2 NWs can be used as a stable catalyst for DMC (Supplementary Fig. 9 ). 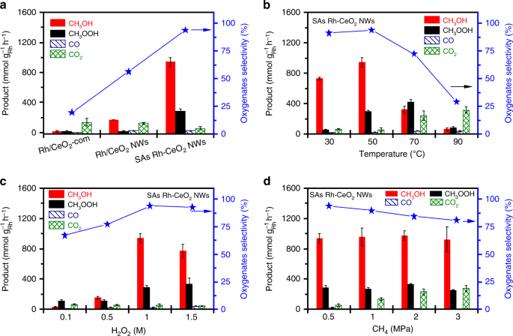Fig. 2: DMC performance on different catalysts. aThe yield and selectivity of oxygenates from Rh/CeO2-com, Rh/CeO2NWs, and SAs Rh-CeO2NWs. Reaction conditions:PCH4: 0.5 MPa, H2O2: 20 mL (1 M),T: 50 °C, reaction time: 1 h, and catalyst weight: 10 mg.bDMC performance at different temperatures over SAs Rh-CeO2NWs. Reaction conditions:PCH4: 0.5 MPa, H2O2: 20 mL (1 M),T: 30-90 °C, reaction time: 1 h, and catalyst weight: 10 mg.cDMC performance at different H2O2concentrations over SAs Rh-CeO2NWs. Reaction conditions:PCH4: 0.5 MPa, H2O2: 20 mL (0.1–1.5 M),T: 50 °C, reaction time: 1 h, and catalyst weight: 10 mg.dDMC performance at different CH4partial pressure over SAs Rh-CeO2NWs. Reaction conditions:PCH4: 0.5–3 MPa, H2O2: 20 mL (1 M),T: 50 °C, reaction time: 1 h, and catalyst weight: 10 mg. The error bars are defined as standard deviation of three experiments. Moreover, to the best of our knowledge, the current DMC performance has outperformed the reported catalysts (Supplementary Table 2 ), suggesting that SAs Rh-CeO 2 NWs can be used as a highly efficient catalyst for DMC to oxygenates under mild conditions. Fig. 2: DMC performance on different catalysts. a The yield and selectivity of oxygenates from Rh/CeO 2 -com, Rh/CeO 2 NWs, and SAs Rh-CeO 2 NWs. Reaction conditions: P CH4 : 0.5 MPa, H 2 O 2 : 20 mL (1 M), T : 50 °C, reaction time: 1 h, and catalyst weight: 10 mg. b DMC performance at different temperatures over SAs Rh-CeO 2 NWs. Reaction conditions: P CH4 : 0.5 MPa, H 2 O 2 : 20 mL (1 M), T : 30-90 °C, reaction time: 1 h, and catalyst weight: 10 mg. c DMC performance at different H 2 O 2 concentrations over SAs Rh-CeO 2 NWs. Reaction conditions: P CH4 : 0.5 MPa, H 2 O 2 : 20 mL (0.1–1.5 M), T : 50 °C, reaction time: 1 h, and catalyst weight: 10 mg. d DMC performance at different CH 4 partial pressure over SAs Rh-CeO 2 NWs. Reaction conditions: P CH4 : 0.5–3 MPa, H 2 O 2 : 20 mL (1 M), T : 50 °C, reaction time: 1 h, and catalyst weight: 10 mg. The error bars are defined as standard deviation of three experiments. Full size image Mechanistic studies on DMC In order to study the mechanism of CH 4 selective oxidation on SAs Rh-CeO 2 NWs, DMC was performed using O 2 as the oxidant to replace H 2 O 2 . 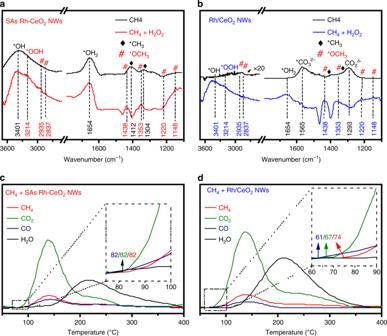Fig. 3: In situ CH4-DRIFTS and CH4-TPSR measurement. a,bIn situ CH4-DRIFTS measurements on SAs Rh-CeO2NWs (a) and Rh/CeO2NWs (b).c,dCH4-TPSR measurements on SAs Rh-CeO2NWs (c) and Rh/CeO2NWs (d). 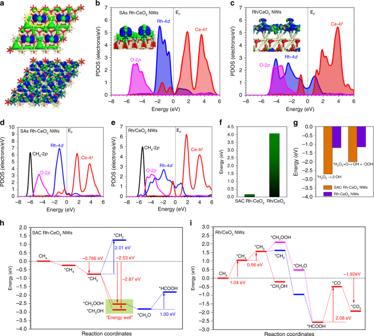Fig. 4: DFT calculations of DMC reaction paths on SAs Rh-CeO2NWs and Rh/CeO2NWs. aThe real spatial contour plots for bonding and antibonding orbitals near EFfor SAs Rh-CeO2NWs and Rh/CeO2NWs.bThe PDOS of SAs Rh-CeO2NWs surface.cThe PDOS of Rh/CeO2NWs surface.dThe PDOS of CH4adsorption on SAs Rh-CeO2NWs surface.eThe PDOS of CH4adsorption on Rh/CeO2NWs surface.fEnergy comparison of [O] desorption from CeO2on SAs Rh-CeO2NWs and Rh/CeO2NWs.gThe reaction energy comparison of generating radicals.hReaction paths and energy profile of DMC over SAs Rh-CeO2NWs.iReaction paths and energy profile of DMC over the Rh/CeO2NWs. As depicted in Supplementary Table 3 , the selectivity of oxygenates is 5.9% when O 2 is solely used as the oxidant, which significantly increases to 92.8% after the addition of 10 μmol H 2 O 2 . Correspondingly, the yield of oxygenates increases from 17.6 to 1159.4 mmol g Rh −1 h −1 , indicating that H 2 O 2 can significantly promote DMC to oxygenates. Based on the previous reports [10] , we speculated that the DMC in the presence of H 2 O 2 might follow radical-triggered reaction paths. Therefore, electron paramagnetic resonance (EPR) was performed to detect the radicals in the present reaction system by using 5,5′-dimethyl-1-pyrroline-N-oxide (DMPO) as the radical scavenger. In order to label the radicals, two contrast experiments were performed in the systems of DMPO + H 2 O 2 + Fe 2+ and DMPO + H 2 O 2 + Fe 2+ + CH 3 OH (detailed information has been given in the experimental section). As shown in Supplementary Fig. 10 , a four-line EPR spectrum with a relative peak ratio of 1:2:2:1 is obtained from the DMPO + H 2 O 2 + Fe 2+ system (Supplementary Fig. 10 , green curve), which can be assigned to ∙OH radical [26] . For the system of DMPO + H 2 O 2 + Fe 2+ + CH 3 OH, a six-line EPR spectrum is recorded, which can be indexed as the characteristic peaks of ∙CH 3 radical (Supplementary Fig. 10 , blue curve) [26] . When DMPO is added into the reaction system, some new peaks of ∙OOH appear in the EPR spectrum in addition to those peaks of ∙CH 3 and ∙OH radicals (Supplementary Fig. 10 , red curve) [27] . The presence of ∙CH 3 , ∙OOH, and ∙OH radicals in the reaction system further confirms that the DMC on the SAs Rh-CeO 2 NWs in H 2 O 2 solution is triggered by radicals. To further study the working mechanism of the radical-triggered DMC on SAs Rh-CeO 2 NWs, in situ DRIFTS measurements were performed to analyze the surface species on SAs Rh-CeO 2 NWs and Rh/CeO 2 NWs when they were exposed to H 2 O 2 and CH 4 . First, we exposed SAs Rh-CeO 2 NWs and Rh/CeO 2 NWs into H 2 O 2 . As shown in Supplementary Fig. 11 , three intense peaks are observed at 3401, 3214, and 1654 cm −1 in the spectra of SAs Rh-CeO 2 NWs and Rh/CeO 2 NWs, which can be assigned to * OH, * OOH, and * OH 2 , respectively [28] . Based on the observations in EPR spectra (Supplementary Fig. 10 ) and previous reports, we conclude that H 2 O 2 can decompose into active radicals on CeO 2 NWs [29] , [30] . When the SAs Rh-CeO 2 NWs are exposed to CH 4 , the characteristic bands of * CH 3 appear at 1412 and 1304 cm −1 (see ref. [31] ), indicating that SAs Rh-CeO 2 NWs can selectively activate CH 4 into * CH 3 (Fig. 3a , black curve). Moreover, two additional bands are observed at 1635 and 3401 cm −1 , which can be ascribed as * OH 2 and * OH, respectively, suggesting that * OH may combine with H from CH 4 decomposition to form * OH 2 . When SAs Rh-CeO 2 NWs are exposed to the mixture of CH 4 and H 2 O 2 (Fig. 3a , red curve), new peaks appear at 2935, 2837, 1438, 1353, 1220, and 1148 cm −1 in the spectrum, which can be assign to the C−H asymmetric stretching vibration, C−H symmetric stretching vibration, CH 3 scissoring vibration, CH 3 asymmetric rocking vibration, C−O stretching vibration and CH 3 symmetric rocking vibration of * OCH 3 , respectively [32] , [33] . The appearance of * OCH 3 , * OH, and * OOH demonstrates the formation of CH 3 OH and CH 3 OOH. By contrast, when Rh/CeO 2 NWs are exposed to CH 4 , only two strong bands of CO 3 2− and * CO 2 δ- are observed at 1589 and 1293 cm −1 (Fig. 3b , black spectrum) [34] . The absence of * CH 3 , * OH, and * OH 2 suggests that CH 4 is overoxidized into CO x species. When Rh/CeO 2 NWs are exposed to the mixture of CH 4 and H 2 O 2 , the intense band of CO 3 2− in the spectrum implies that CO x are the dominate products despite the appearance of * OCH 3 and * OH bands (Fig. 3b , blue curve) [35] , which is consistent with our experimental results (Fig. 2a ). Fig. 3: In situ CH 4 -DRIFTS and CH 4 -TPSR measurement. a , b In situ CH 4 -DRIFTS measurements on SAs Rh-CeO 2 NWs ( a ) and Rh/CeO 2 NWs ( b ). c , d CH 4 -TPSR measurements on SAs Rh-CeO 2 NWs ( c ) and Rh/CeO 2 NWs ( d ). Full size image To further confirm the activation of CH 4 on Rh, CH 4 temperature programmed surface reaction (TPSR) was performed to investigate the CH 4 conversion on CeO 2 NWs, SAs Rh-CeO 2 NWs, and Rh/CeO 2 NWs. No obvious peaks are observed in the TPSR pattern of CeO 2 NWs, suggesting that CeO 2 NWs are inactive for CH 4 activation under the indicated conditions (Supplementary Fig. 12 ). When CH 4 -TPSR measurements were performed on SAs Rh-CeO 2 NWs and Rh/CeO 2 NWs, the peaks of CH 4 , CO, CO 2 , and H 2 O appear in TPSR patterns, suggesting that Rh atoms play as the active sites for CH 4 activation (Fig. 3c, d ), which is in good agreement with results from the in situ DRIFTS measurement (Fig. 3a, b ). Despite the appearance of peaks in TPSR patterns, the different onset temperatures ( T onset ) suggest that the reaction paths are different on SAs Rh-CeO 2 NWs and Rh/CeO 2 NWs (Fig. 3c, d ). For SAs Rh-CeO 2 NWs, the T onset of CH 4 (~82 °C, formed via * CH 3 hydrogenation) is closed to that of CO (~82 °C) and CO 2 (~82 °C), indicating that * CH 3 hydrogenation (to form CH 4 ) and overdehydrogenation (to form CO x ) competitively occur on the SAs Rh-CeO 2 NWs. By contrast, the T onset of CO 2 (~67 °C) and CO (~61 °C) is significantly lower than that of CH 4 (~74 °C) in TPSR patterns of Rh/CeO 2 NWs, indicating that overoxidation for the formation of CO and CO 2 is preferential [5] . DFT calculations Finally, DFT calculations were performed to reveal the reaction paths of CH 4 oxidation on SAs Rh-CeO 2 NWs and Rh/CeO 2 NWs. The real spatial orbital distribution apparently shows the concentrated electron-rich feature on SAs Rh, which indicates the Rh site possesses a superior reaction priority among the available sites on the surface. Meanwhile, Rh cluster on CeO 2 shows widely separated electronic distribution over the surface, which shows the disperse electroactive region (Fig. 4a ). The projected density of states (PDOS) support that the highly concentrated electronic activity of SAs Rh on the surfaces is attributed to the sharp Rh-4d occupation near the Fermi level (E F ). The Ce-4f bands mainly locate above E F , while O-2p bands concentrate on E v − 4.5 eV. The evident coupling between Rh-4d and Ce-4d confirms the stabilization of SAs Rh by the protection of bottom Ce (Fig. 4b ). In comparison, the Rh-4d bands become much broad in Rh/CeO 2 , covering from E v − 5.0 eV E v + 2.0 eV. The evident match among Rh-4d bands and O-2p bands and Ce-4f bands indicates a strong coupling between the surface Rh cluster and bottom CeO 2 (Fig. 4c ). The electronic structures of CH 4 adsorption are further presented to illustrate the different activity toward the DMC process. It is noted the dominant peak of Rh-4d in SAs Rh-CeO 2 upshifts from E v − 2.0 eV toward E v − 1.0 eV due to the electron transfer with CH 4 (Fig. 4d ). Meanwhile, the close distance between Rh-4d bands and O-2p bands on Rh/CeO 2 NWs demonstrates the strong couplings between CH 4 and local O atoms, which lead to the over-binding effect with increased energy barriers for the consecutive dehydrogenation of CH 4 (Fig. 4e ). Fig. 4: DFT calculations of DMC reaction paths on SAs Rh-CeO 2 NWs and Rh/CeO 2 NWs. a The real spatial contour plots for bonding and antibonding orbitals near E F for SAs Rh-CeO 2 NWs and Rh/CeO 2 NWs. b The PDOS of SAs Rh-CeO 2 NWs surface. c The PDOS of Rh/CeO 2 NWs surface. d The PDOS of CH 4 adsorption on SAs Rh-CeO 2 NWs surface. e The PDOS of CH 4 adsorption on Rh/CeO 2 NWs surface. f Energy comparison of [O] desorption from CeO 2 on SAs Rh-CeO 2 NWs and Rh/CeO 2 NWs. g The reaction energy comparison of generating radicals. h Reaction paths and energy profile of DMC over SAs Rh-CeO 2 NWs. i Reaction paths and energy profile of DMC over the Rh/CeO 2 NWs. Full size image Since EPR and in situ DRIFTS results show that lattice O atoms of CeO 2 are feasibly bonded with H in H 2 O 2 . From the energetic view, DFT also proves the superior flexibility of O in SAs Rh-CeO 2 NWs with only 0.16 eV energy barrier. Due to the steric hindrance from the surface coverage of Rh cluster, the energy barrier of the detachment of O in Rh/CeO 2 NWs increases to 4.06 eV, demonstrating a slow efficiency of generating ∙OOH radicals (Fig. 4f ). The further reaction energies also support that the generations of both ∙OH and ∙OOH radicals are much more preferred in SAs Rh-CeO 2 NWs, satisfying the prerequisite of radical-mediated DMC process (Fig. 4g ). The SAs Rh-CeO 2 NWs deliver an overall downhill trend to the formation final product CH 3 OH and CH 3 OOH, representing a high electronic activity. The spontaneous adsorption of CH 4 and facile C−H bond cleavage indicates the fast activation of C−H bond, which leads to the efficient DMC process. Particularly, the further reaction of CH 3 OOH toward HCOOH has been suppressed by the high energetic barrier of 1 eV, guaranteeing the reaction locking for desired products. The formation of CH 3 OH releases 2.87 eV, which is slightly larger energy than that of CH 3 OOH (2.53 eV), explaining the higher yield of oxygenates in our experiments. Meanwhile, the high energy cost (2.01 eV) to achieve further C−H bond cleavage of CH 3 facilitates the high selectivity of DMC on the SAs Rh-CeO 2 NWs (Fig. 4h ). In contrast, the activation of C−H bond in CH 4 faces stepped energy barriers toward * CH 2 on Rh/CeO 2 NWs, indicating a much lower selectivity of oxygenates. The formation of CH 3 OOH induced by the ∙OOH radical requires an energy cost of 0.47 eV, while the generation of CH 3 OH is energetically favorable. Notably, both * CH 2 and CH 3 OOH exhibit an evident energy drop toward the formation of HCOOH, indicating that the overoxidation of CH 4 is preferred. However, the further oxidation of HCOOH to CO shows an energy barrier of 2.08 eV, which further lowers the DMC efficiency. The overall energy release is 1.92 eV, which is much smaller than that of SAs Rh-CeO 2 NWs, supporting the stronger reaction activity of SAs Rh-CeO 2 NWs toward the DMC conversion (Fig. 4i ). Reaction pathways Combining the results from EPR, in situ DRIFTS and DFT calculations, we thus summarized the reaction paths of DMC on the SAs Rh-CeO 2 NWs and Rh/CeO 2 NWs (Supplementary Figs. 13 and 14 ). As displayed in Supplementary Fig. 13 , for the SAs Rh-CeO 2 NWs, H 2 O 2 can decompose into ∙OH on two neighboring Ce (III) atoms (step 1). On the other hand, H 2 O 2 can decompose into ∙OOH on Ce (IV), and the remaining ∙H will combine with [O] (lattice O of CeO 2 ) connected with the Ce (IV) in CeO 2 NWs to form ∙[O]H (step 2). The adsorbed CH 4 on Rh SA can be oxidized into ∙CH 3 and H 2 O with the assistance of ∙OH (step 3). As a result, the formed ∙CH 3 will react with the ∙OOH and ∙[O]H radicals to produce CH 3 OOH and CH 3 [O]H via steps 4 and 5. It should be noted that the lattice [O] in CeO 2 NWs will be compensated by H 2 O 2 (Ce (III) → Ce (IV)). By contrast, the reaction paths are different on the Rh/CeO 2 NWs, despite the paths of H 2 O 2 decomposition (steps 1−2) are the same (Supplementary Fig. 14 ). On Ru clusters, CH 4 can be activated into ∙CH 3 by ∙OH, which may (i) react with ∙[O]H to CH 3 [O]H (step 4), or (ii) combine with ∙OOH to produce CH 3 OOH (step 5), or (iii) be further oxidized into * CH 2 by ∙OH (step 6). Both the CH 3 OOH and * CH 2 will be converted into * CH 2 O (steps 7 and 8) and then to * HCOOH on the Rh/CeO 2 NWs (step 9). Finally, HCOOH will be further oxidized into CO x in the presence of ∙OH (steps 10−11). In summary, we demonstrated that SAs Rh-CeO 2 NWs can be used for DMC to oxygenates. Compared with the low selectivity (56.4%) and yield (189.4 mmol g Rh −1 h −1 ) of oxygenates from Rh/CeO 2 NWs, the selectivity and yield of CH 3 OH and CH 3 OOH are 93.9% and 1231.7 mmol g Rh −1 h −1 on SAs Rh-CeO 2 NWs at 50 °C, which to the best of our knowledge outperforms the reported values in the literatures. In situ characterizations and experiments were performed to study the mechanism. It is shown that CeO 2 NWs play a vital role in the generation of ∙OH and ∙OOH radicals, which can significantly promote the oxidation of CH 4 via different reaction paths. To be more specific, SAs Rh-CeO 2 NWs can selectively activate CH 4 to * CH 3 , leading to the formation of oxygenate in the presence of H 2 O 2 , while Rh/CeO 2 NWs favor the overoxidation of CH 4 to form CO x , leading to a low selectivity and yield of oxygenates. DFT calculations reveal the facile C−H bond activation and reaction locking on SAs Rh-CeO 2 NWs guarantees the high selectivity and yield of DMC, supplying solid evidence for experimental results. This work may not only provide a highly active and selective catalyst for DMC to oxygenate but also promote the researches of SACs in heterogeneous catalysis. Preparation of CeO 2 nanowires (NWs) and SAs Rh-CeO 2 NWs In a typical preparation of CeO 2 NWs, 12 mL CeCl 3 (0.5 mmol, Alfa Aesar) and sodium oleate (0.75 mmol, Tokyo Chemical Industry) aqueous solution were added into a 20-mL Teflon-lined stainless-steel autoclave. The mixture was magnetically stirred at 800 rpm (round per minute) for 0.5 h. To this solution, n -butylamine (1 mL, Sinopharm) was slowly added into the solution under stirring for another 0.5 h. Afterward, the autoclave was heated at 160 °C for 10 h before it was cooled to room temperature. The resulting products were collected by centrifugation and washed three times with cyclohexane/acetone mixture, and then dried at room temperature overnight. The powder products were subjected to thermal annealing in an air atmosphere at 400 °C for 10 min at a heating rate of 10 °C min −1 . For SAs Rh-CeO 2 NWs, all the parameters were the same with CeO 2 NWs, except for adding extra Na 3 RhCl 6 (5 μmol, Aldrich). Preparation of Rh/CeO 2 NWs and Rh/CeO 2 -com The Rh/CeO 2 NWs and Rh/CeO 2 -com were prepared via a conventional wet-impregnation method. Typically, a certain amount of Na 3 RhCl 6 solution was dropwise added into the as-prepared CeO 2 NWs and commercial CeO 2 (99.9%, Inoke) under moderate stirring. The resultant slurry was mixed evenly and then dried in an oven at 80 °C overnight, and then subjected to thermal annealing in air at 400 °C for 10 min at a heating rate of 10 °C min −1 . Finally, the calcinated samples were re-washed water for three times via centrifugation, and then dried at 100 °C overnight. Characterization The morphologies and sizes of the NWs were determined by TEM (Hitachi, HT7700) at 120 kV. AC-HAADF-STEM images were taken on JEM-ARM200F with a cold-field emission gun and a spherical aberration corrector. The Rh loading amounts were determined by the inductively coupled plasma atomic emission spectroscopy (ICP-AES) (710-ES, Varian). XRD patterns were collected on X’Pert-Pro MPD diffractometer (Netherlands PANalytical) with a Cu Kα X-ray source ( λ = 1.540598 Å). XPS was done with an SSI S-Probe XPS Spectrometer. The carbon peak at 284.6 eV was used as a reference to correct for charging effects. The X-ray absorption data at the Rh K-edge of the samples were recorded at room temperature in transmission mode using ion chambers at beamline BL14W1 of the Shanghai Synchrotron Radiation Facility (SSRF), China. The station was operated with a Si (311) double-crystal monochromator. During the measurement, the synchrotron was operated at energy of 3.5 GeV and a current between 150 and 210 mA. The photon energy was calibrated with the first inflection point of Rh K-edge in Rh metal foil. Typical process for selective oxidation of CH 4 The selective oxidation of CH 4 was performed in a 60-mL stainless-steel autoclave. Typically, 20 mL H 2 O 2 solution (1 M) and 10 mg of catalyst were added into a Teflon inlet. Afterward, the autoclave was pressurized with CH 4 (0.5 MPa). The reaction was performed at 50 °C with stirring at 800 rpm for 1 h. In our work, we used a commercial Agilent GC integrated system with a flame ionization detector (FID) for the detection of gaseous products. This system contains three columns (two hayesep Q columns and one 5 A mol sieve column) for the separation of gaseous products. Both CO and CO 2 were converted into CH 4 via a methanator to analyze by FID. All the gaseous products were introduced into two tandem hayesep Q columns for pre-separation. CO 2 was completely separated in this process and introduced into the FID via a switch valve. The remaining gases were further introduced into a 5 A mol sieve column for further separation. 1 H nuclear magnetic resonance spectroscopy ( 1 H-NMR, Bruker 600 MHz) was employed for structural analysis of liquid products, in which dimethylsulfoxide (DMSO, 1‰) and deuteroxide were used as the internal standard and solvent, respectively. The liquid products were analyzed by a gas chromatograph (Persee G5) with a FID using a KB-5 column. In total, 10 μL of isopropanol/H 2 O (1%) was used as the internal standard adding into 1 mL reaction mixture for analyzing CH 3 OH and CH 3 OOH. The amount of CH 3 OH was calculated using the standard curve method. Afterward, CH 3 OOH was converted to CH 3 OH using hydrazine hydrate (0.1 mL). The total amount of CH 3 OH and CH 3 OOH were analyzed by gas chromatograph, and the amount of CH 3 OOH was obtained by minusing. For each catalytic test, error bar was obtained by repeating three times. The yields of products and the selectivity were calculated using Eqs. ( 1 ) and ( 2 ). Yields of products ( mmol g_Rh^ - 1 h^ - 1) = mmol of products/g of Rh/h of reaction time
 (1) 
    Oxygenates selectivity ( %) = 	  mmol of ( CH_3OOH  + CH_3OH) 
    × 100/mmol of all products
 (2) EPR measurement The detection of free radicals in the reaction process of DMC was performed at a JEOL JES-FA200 electron paramagnetic resonance spectroscopy (EPR, 9.062 GHz), using DMPO as the scavenger. Typically, 1 mL DMPO-H 2 O (100 mmol L −1 ) was added into 1 mL of reaction mixture. The mixed solution was immediately transferred to a capillary tube (diameter: 0.1 mm; filling liquid height: ~5 cm), which was then fixed in the resonant cavity of the spectrometer. EPR measurements were detected at room temperature and recorded by three scans. The contrast experiments were performed to determine the type of radicals by characteristic peaks. Contrast experiment 1 (labeled as DMPO + H 2 O 2 + Fe 2+ ): 1 mL ferrous (II) sulfate (FeSO 4 , 50 mmol L −1 ) and nitric acid solution (pH = 4) were mixed with 1 mL DMPO-H 2 O (100 mmol L −1 ) under moderate stirring for 2 min, followed by adding 50 μL of H 2 O 2 (30 wt.%). Contrast experiment 2 (labeled as DMPO + H 2 O 2 + Fe 2+ + CH 3 OH): all the processes were the same with contrast experiment 1, except for the addition of 1 mL of CH 3 OH (100 mmol L −1 ) into the solution. CO-DRIFTS measurement In all, 20 mg sample was packed into a Harrick Praying Mantis high-temperature reaction chamber (CaF 2 windows) mounted inside of a Thermo Scientific Praying Mantis diffuse reflectance adapter, set inside of a Thermo Scientific Nicolet 6700 Fourier transform infrared (FT-IR) spectrometer using liquid nitrogen cooled mercury–cadmium–telluride detector (MCT). Gases were flowed to the reaction chamber using Alicat mass flow controllers. Prior to CO-DRIFTS measurement, the sample was pretreated by heating in CO/Ar (10 vol.%) flow (50 mL min −1 ) at different temperatures (e.g., −30 °C, 50 °C, and 150 °C), followed by flushing with Ar flow (50 mL min −1 ) for 1 h. After cooling to −30 °C in the same Ar flow, CO/Ar (10 vol.%, 50 mL min −1 ) was flowed through the sample at −30 °C for 0.5 h. Finally, the sample was flushed with Ar flow (50 mL min −1 ) at −30 °C for 0.5 h to remove the physically adsorbed CO on the surface sample. The CO-DRIFTS spectra were obtained by averaging 16 sequentially collected scans at a resolution of 4 cm −1 . In situ CH 4 -DRIFTS measurement For in situ CH 4 -DRIFT, 20 mg sample was packed into a Harrick Praying Mantis high-temperature reaction chamber (CaF 2 windows) mounted inside of a Thermo Scientific Praying Mantis diffuse reflectance adapter, set inside of a Thermo Scientific Nicolet 6700 FT-IR spectrometer using liquid nitrogen cooled MCT detector. The sample was pretreated by heating in Ar flow (50 mL min −1 ) at 400 °C for 1 h and cooled down to 50 °C in the same Ar flow. Gases (5 vol.% CH 4 /Ar or Ar) were flowed using Alicat mass flow controllers. The hydrogen peroxide is brought into the chamber by a carrier gas (5 vol.% CH 4 /Ar) with a positive pressure (0.15 MPa). Afterward, 5 vol.% CH 4 /Ar with the hydrogen peroxide was flowed through the catalyst bed at 50 °C for 0.5 h, followed by flushing with Ar flow (50 mL min −1 ) for 0.5 h at the same temperature. The in situ CH 4 -DRIFTS spectra were obtained by averaging 16 sequentially collected scans at a resolution of 4 cm −1 . For CH 4 -DRIFTS measurement, all the parameters are the same with in situ CH 4 -DRIFTS measurement, except for the absence of H 2 O 2 . DFT calculations All calculations were carried out using DFT implemented in the CASTEP [36] . The electron exchange and correlation interaction were calculated with the generalized gradient approximation (GGA) in the parametrization of Perdew–Burke–Ernzerhof (PBE) pseudopotentials [37] , [38] . To minimize the computational cost for the surface modeling, ultrasoft pseudopotential scheme has been chosen with the cutoff energy of 410 eV [39] , [40] . For both SAs Rh-CeO 2 and Rh/CeO 2 , the CeO 2 crystal has been cleaved along the (111) plane with three-layer thickness. For SAs Rh-CeO 2 model, only one Rh atom is deposited onto the CeO 2 surface within the unit cell to demonstrate the single-atom catalyst. For Rh/CeO 2 NWs model, the Rh cluster consists of eight atoms, which is cleaved from the bulk Rh crystal along the (111) plane. We imposed a 15 Å vacuum space along z -direction to supply sufficient space for the adsorption behaviors without interactions between lattice. For all the geometry optimizations, the Hellmann–Feynman forces will be converged to <0.001 eV/A, while the total energy has been converged to 5 × 10 −5 eV per atom. The coarse k-point has been applied for the energy minimization based on the Broyden–Fletcher–Goldfarb–Shannon (BFGS) algorithm [41] , [42] .